Room-temperature exciton coherence and dephasing in two-dimensional nanostructures Electronic coherence has attracted considerable attention for its possible role in dynamical processes in molecular systems. However, its detection is challenged by inhomogeneous line broadening and interference with vibrational coherences. In particular, reports of ‘persistent’ coherent exciton superpositions at room temperature remain controversial, as the related transitions give typically shorter optical dephasing times of about 10–20 fs. To rationalize these reported long-lived coherences, several models have been proposed, involving strong correlation in the mechanisms of decoherence or that electronic coherences may be sustained by resonant vibrational modes. Here we report a decisive example of electronic coherence occurring in a chemical system in a ‘warm and wet’ (room-temperature solution) environment, colloidal semiconductor nanoplatelets, where details are not obscured by vibrational coherences nor ensemble dephasing. Comparing the exciton and optical coherence times evidences a partial correlation of fluctuations underlying dephasing and allows us to elucidate decoherence mechanisms occurring in these samples. Dynamical chemical processes in solution are generally regarded as proceeding incoherently from initial to final states. Therefore, the initial report of Engel et al . [1] stimulated great interest, because it proposes that electronic coherences may play a role in the efficiency of energy transfer occurring in biological processes. Subsequent work includes discoveries of coherence in light harvesting at ambient temperature [2] , [3] , conjugated polymers [4] and supramolecular complexes [5] . The study of electronic coherences has been encouraged by the application of new ultrafast techniques such as two-dimensional (2D) spectroscopy. However, it is often difficult to examine electronic coherence and its intrinsic dephasing in complex systems when mean energy gaps in the ensemble are disordered. This inhomogenous broadening results in an apparent shortening of the observed ensemble coherences called ‘fake decoherence’ [6] , [7] . Moreover, the presence of numerous vibrational modes in molecular chromophores [8] and even the (nonresonant) solvent [9] makes interpretation of the coherent signals in time-resolved experiments particularly challenging. To try to circumvent these complexities, analyses of oscillation amplitudes in 2D maps have been developed [10] . However, even when isolated, the nature of the coherent signal itself is still debated [11] , [12] . The observation of electronic coherences that survive markedly longer than optical coherences between the ground states and excited states (given by the transition natural linewidth) was first explained by invoking a strong correlation in the energy fluctuations of the two electronic levels [1] , [3] , [13] , [14] . In that case, the amplitude of energy gap fluctuations is very small, preserving the coherent superposition. More recently, models were proposed where the electronic coherence is sustained by interaction with a resonant vibrational mode [14] , [15] , [16] . To clarify and perhaps unify the theories proposed for the observation of electronic coherences lasting for hundreds of femtoseconds, model systems are required wherein inhomogeneous broadening is negligible and electronic coherences can be clearly distinguished from their vibrational counterparts. In this report, we use 2D electronic spectroscopy (2DES) to study the exciton superposition and dephasing in colloidal nanoplatelets (NPLs) at room temperature. The NPLs turn out to be ideal systems for studying electronic coherence owing to their narrow spectral lineshapes and absence of ensemble disorder. Therefore, a direct comparison between optical coherence and excitonic coherence dephasing times is possible. A partial correlation in the fluctuations of the two excited states is revealed and explains how the coherence can be observed for up to ~100 fs at room temperature. However, the time scale of the exciton superposition remains in the same order of magnitude than of the optical coherence between the ground and excited states due to the presence of uncorrelated dephasing pathways. Here we show that this limiting pathway is not related to the exciton relaxation, in contrast to what has been suggested in previous studies. Sample characterizations Colloidal NPLs are anisotropic semiconductor nanostructures with optical spectra characteristic of quasi-2D excitons [17] . In this report, we mainly compare CdSe NPLs with a thickness of five monolayers (1.5 nm, NPL550) and their corresponding CdSe/CdZnS heterostructure, with a shell of ~2 nm (NPLcs550) [18] . The high aspect ratio of these 2D nanostructures is evident in the transmission electron micrographs shown in Fig. 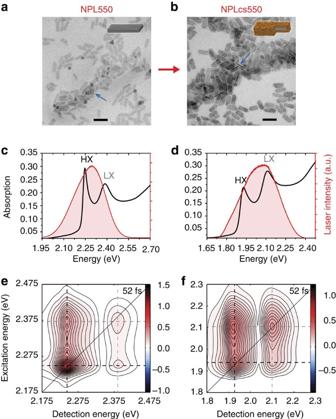Figure 1: Nanoplatelet structure and spectroscopy. (a,b) Transmission electron microscopy pictures of the atomically flat CdSe NPL550 (a) and of the corresponding heterostructure NPLcs550 (b) with shell inhomogeneities (schematics in inset). Scale bars, 50 nm. The blue arrows emphasize the 2D shape of the samples by pointing NPLs standing on their edge. Absorption spectra of CdSe (c, black line) and CdSe/CdZnS (d, black line) NPLs showing the HX and LX exciton transitions. The typical laser spectra used in the 2D experiments to cover the green and orange ranges are shown in red incandd, respectively. (e,f) Representative 2DES spectra (total and magnitude signal) for a waiting timeT=52 fs. The well-resolved diagonal peaks are located at the excitation and detection energies of HX and LX (black and grey dashed lines, respectively). 1a,b , respectively (measured sizes, Supplementary Table 1 ). The room-temperature absorption spectra ( Fig. 1c,d ) show well-defined transitions of bound excitons present due to the strong quantum one-dimensional confinement [17] . The two first absorption peaks arise from electronic transitions involving different hole bands and are labelled heavy-hole and light-hole excitons (HX and LX, respectively) [17] . These peaks show an increase of the HX–LX splitting, a broadening and a notable red shift during the CdZnS shell growth characteristic of a change in the wavefunction delocalization. Figure 1: Nanoplatelet structure and spectroscopy. ( a , b ) Transmission electron microscopy pictures of the atomically flat CdSe NPL550 ( a ) and of the corresponding heterostructure NPLcs550 ( b ) with shell inhomogeneities (schematics in inset). Scale bars, 50 nm. The blue arrows emphasize the 2D shape of the samples by pointing NPLs standing on their edge. Absorption spectra of CdSe ( c , black line) and CdSe/CdZnS ( d , black line) NPLs showing the HX and LX exciton transitions. The typical laser spectra used in the 2D experiments to cover the green and orange ranges are shown in red in c and d , respectively. ( e , f ) Representative 2DES spectra (total and magnitude signal) for a waiting time T =52 fs. The well-resolved diagonal peaks are located at the excitation and detection energies of HX and LX (black and grey dashed lines, respectively). Full size image 2D electronic spectroscopy 2DES enables us to study the ultrafast dynamics and, more specifically, temporal evolution of coherences produced by photo-excitation. The third-order radiated signal resulting from the interaction of the sample with three broadband femtosecond pulses is heterodyne detected and recorded as a function of the pump–probe delay time T (waiting time). For each T , we plot a 2D map of the signal amplitude as a function of the detection energy and of the excitation energy (see Supplementary Method ). The latter axis is retrieved through Fourier transformation of the signal along the time dimension corresponding to the first coherence time [19] , τ ( Supplementary Fig. 1 ). The evolution of the peaks in amplitude and shape reveals information about the dynamics of the system and its interaction with the environment [20] , [21] . 2D map and spectral lineshape 2DES has previously revealed information about excitons in quantum wells, the epitaxial equivalent of NPLs, with samples maintained at cryogenic temperature [22] , [23] . Griffin et al . [24] have recently reported a 2DES study of colloidal CdSe NPLs at room temperature, but weak overlap between the laser spectrum and the higher-energy transition mostly limited the study to the HX dynamics. 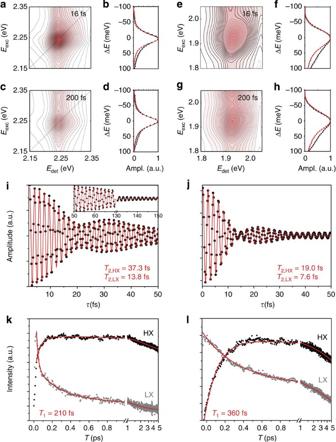Figure 2: HX spectral lineshapes with optical coherences and exciton relaxation. Magnitude rephasing 2DES spectra zoomed into the lower diagonal peak of CdSe NPLs (a,c) and CdSe/CdZnS NPLs (e,g) for the waiting timesTindicated. The absence of ensemble broadening is highlighted by comparing the diagonal and anti-diagonal lineshapes (black squares and red dots, respectively) extracted from theaandeat earlyTtime (plotsb,f) and fromc,gat longer time (plotsd,h). (i,j) Evolution of the amplitude of the third-order signal of CdSe (i) and CdSe/CdZnS (j) NPLs along the first coherence timeτ(rephasing part and black dots) at HX detection energy. The signals were fitted with a sum of damped sine functions corresponding to HX and LX frequencies (red lines). The dephasing timesT2,HXandT2,LXare displayed in both cases. (k,l) Pump–probe measurements at HX (black dots) and LX (grey dots) detection energies for CdSe NPLs (k) and the corresponding heterostructure (l). The semi-log scale was chosen to emphasize the early time rise of HX population and the additional decay of LX population corresponding to the exciton relaxation. The decays/growths are fitted with exponential functions (red lines) and the extracted relaxation timesT1are displayed in both cases. Here we study CdSe and CdSe/CdZnS NPLs by 2DES with 9–13 fs duration pulses ( Supplementary Figs 2 and 3 , and Supplementary Table 2 ) that cover the two first excitonic transitions ( Fig. 1c,d ). In Fig. 1e,f , we plot the room-temperature 2D spectrum of the two samples for a waiting time of T =52 fs (total, magnitude signal). Diagonal and cross-peaks are clearly resolved at the four combinations of excitation and detection energies of HX and LX. The presence of the cross-peaks confirms the strong ‘coupling’ between the two transitions expected, because they share the same electron state [17] . By looking at the absorptive spectrum (real part of the total signal after phasing, Supplementary Fig. 4 ), clear negative features are visible at the low detection energy side of the peaks of CdSe NPLs and at the high-energy side for the heterostructure samples. These excited state absorption features are shifted relatively to the bleach features by the biexciton-binding energy. The change of sign of the biexciton-binding energy with the CdZnS shell growth reveals a decrease of the overlap between the electron and hole wavefunctions [25] . The 2DES spectra of the CdSe and CdSe/CdZnS NPLs exhibit notably different spectral lineshapes. In particular, when we zoom in to the low-energy diagonal peak of the 2D spectrum corresponding to the HX transition ( Fig. 2a–h , rephasing magnitude signal), we see that NPL550 has a diamond-shaped peak characteristic of a 2D Lorentzian lineshape ( Fig. 2a,c ), whereas the corresponding heterostructure displays a more round peak shape, characteristic of a 2D Gaussian function ( Fig. 2e,g ). In both cases, the peaks are slightly elongated along the excitation axis, similar to previous reports on epitaxial quantum wells where the elongation was attributed to excitation-induced dephasing effects [26] . The linewidths of the NPL transitions strongly increase with the laser fluence owing to many-body interactions ( Supplementary Fig. 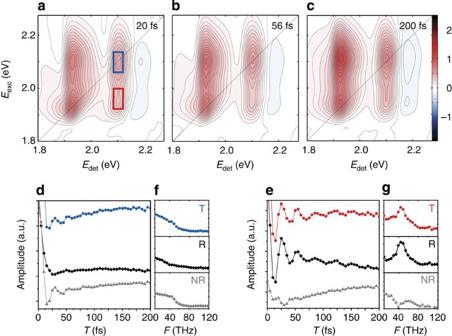Figure 3: Evidence for electronic coherences. (a–c) Absorptive 2DES spectra (total and real signal) of CdSe/CdZnS NPLs at four different waiting times (Tshown in inset). The spectra show no obvious differences, except for the upper cross-peak that grows in time, owing to the LX to HX exciton relaxation. (d,e) The electronic coherences are revealed by quantum beats alongTin the high-energy diagonal peak (d, blue dots) and in the lower cross-peak (e, red dots) of the total signal (T). The oscillations come from the rephasing pulse sequence (R, black diamonds) for the cross-peak, whereas from the non-rephasing one (NR, grey triangles) in the case of the diagonal peak, as expected for pure electronic coherences. All the time traces correspond to an average of three different experimental scans. (f,g) Fourier transforms of the different signals to highlight the frequency spectrum of coherent oscillations. 5 ), and thus experiments were performed at a relatively low pulse energy (50–100 μJ cm −2 , see Supplementary Table 3 and Supplementary Note 1 ). Figure 2: HX spectral lineshapes with optical coherences and exciton relaxation. Magnitude rephasing 2DES spectra zoomed into the lower diagonal peak of CdSe NPLs ( a , c ) and CdSe/CdZnS NPLs ( e , g ) for the waiting times T indicated. The absence of ensemble broadening is highlighted by comparing the diagonal and anti-diagonal lineshapes (black squares and red dots, respectively) extracted from the a and e at early T time (plots b , f ) and from c , g at longer time (plots d , h ). ( i , j ) Evolution of the amplitude of the third-order signal of CdSe ( i ) and CdSe/CdZnS ( j ) NPLs along the first coherence time τ (rephasing part and black dots) at HX detection energy. The signals were fitted with a sum of damped sine functions corresponding to HX and LX frequencies (red lines). The dephasing times T 2,HX and T 2,LX are displayed in both cases. ( k , l ) Pump–probe measurements at HX (black dots) and LX (grey dots) detection energies for CdSe NPLs ( k ) and the corresponding heterostructure ( l ). The semi-log scale was chosen to emphasize the early time rise of HX population and the additional decay of LX population corresponding to the exciton relaxation. The decays/growths are fitted with exponential functions (red lines) and the extracted relaxation times T 1 are displayed in both cases. Full size image The distinct lineshapes reveal differences in the origin of line broadening. Lorentzian peaks are usually characteristic of homogeneous broadening in the fast frequency fluctuation regime. CdSe NPL550 shows similar diagonal and anti-diagonal linewidths for all T times recorded, confirming the absence of ensemble broadening in this sample ( Fig. 2b,d ). This result is in marked contrast to previous 2DES studies of more conventional colloidal nanoparticles [24] , [27] and thus provides further evidence indicating the NPLs are synthesized with a thickness controlled with atomic precision [17] . Gaussian lineshapes generally indicate inhomogeneous broadening, that is, due to a distribution of mean electronic energy gaps throughout the ensemble. This latter case should give an elongated peak along the diagonal in the 2D photon-echo (rephasing) spectrum before spectral diffusion occurs [28] . Nevertheless, despite Gaussian exciton lineshapes, the CdSe/CdZnS NPLcs550—which also clearly show irregularities along the NPL thickness, as seen with the change of contrast in Fig. 1b —have similar diagonal and anti-diagonal linewidths in the 2D spectra ( Fig. 2f,h ). This reveals that the delocalization length of the exciton in the 2D NPL plane at room temperature is larger than the characteristic size of the shell variation [29] , and thus the effective potential felt by the exciton results from an average over the delocalization and is similar from NPL to NPL (exchange narrowing effect [30] , see Supplementary Fig. 6 and Supplementary Note 2 ). The spectral broadening occurring during the shell growth was previously attributed to an increase of the coupling with the longitudinal optical phonons [31] . However, in the same report, an inhomogeneous broadening is revealed at low temperature for the core/shell samples. We propose the larger spectral linewidths of the heterostructures compared with those of the core sample’s result from the interaction of the delocalized excitons with surface defects, as reported for in single-walled carbon nanotubes [32] . In contrast to the HX transition, the LX lineshape is Gaussian shaped in both samples and broader. These lineshapes suggest different dephasing mechanisms for the optical coherence of each of the two transitions. We characterize the optical coherence for HX and LX transition, and determine the corresponding optical dephasing times T 2,HX and T 2,LX . Assuming Lorentzian lineshapes, the radiated signal after the three pulse interactions evolves according to exp(− iω ge τ ) × exp(− τ / T 2,e ), where ω ge is the absorption angular frequency of the electronic transition between the ground state g and the excited state e , and T 2,e is the associated dephasing time (see Supplementary Notes 3 ). We thus plot the amplitude of the third-order signal as a function of coherence time τ , before Fourier transform along the excitation axis ( Fig. 2i,j ). In both samples, a beating envelope modulates the optical frequency oscillations due to the presence of the strong cross-peak. By fitting the coherent signals of CdSe NPLs ( Fig. 2i ), we find T 2,HX =37.3±0.4 and T 2,LX =13.8±0.2 fs. In the case of NPLcs550 ( Fig. 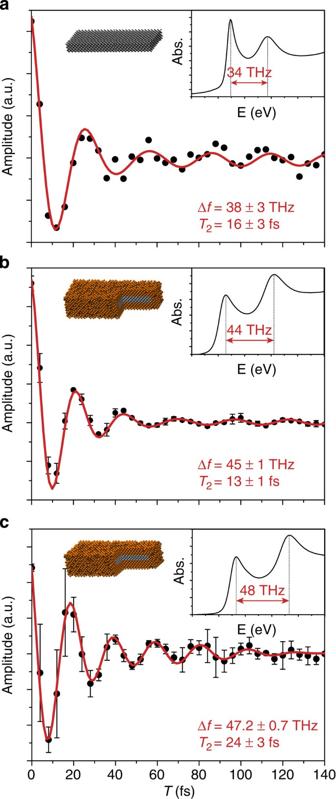Figure 4: Determination of the excitonic coherence dephasing times. (a–c) The amplitude evolutions along the waiting timeTof the lower cross peak of the rephasing 2D spectrum (real part and population relaxation removed) of CdSe NPL550 (a), CdSe/CdZnS NPLcs550 (b) and CdSe/CdZnS NPLcs510 (c) are shown as black dots. The error bars, when displayed, are the s.d. estimated from three different scans. Red lines: fits with two exponentially damped sine functions. Parameters relating to the short decay are shown in red (frequency Δfand dephasing timeT2). For each sample, the HX–LX splitting frequency evident from the absorption spectrum shown in the inset of each panel matches the frequency of the coherent oscillation detected by 2DES. 2j ), T 2,HX =19.0±0.4 and T 2,LX =7.6±0.1 fs ( Supplementary Table 4 ). Exciton relaxation To determine whether the LX to HX relaxation can explain the shorter dephasing time for LX [24] , [33] , we performed pump–probe measurements over an extended time range ( Fig. 2k,l ). The LX to HX exciton relaxation results in a rise of the HX bleach (refill of the HX exciton state) and in an additional decay at the LX bleach (depopulation of the LX state) at early time ( Supplementary Note 4 ). By fitting the signal evolution, we find a relaxation time T 1 ≈210 fs for CdSe NPL550 and longer, about 360 fs, for the corresponding heterostructure (see Supplementary Table 5 ). For each sample, the exciton relaxation time is at least one order of magnitude longer than the dephasing time of the LX optical coherence, and thus cannot be its main source of dephasing. Therefore, we propose that the faster optical dephasing for the LX transition compared with HX arises from coupling of the LX discrete state with the underlying continuum, as was proposed for epitaxial quantum wells [34] , [35] , or with surface states [36] . Exciton coherence Monitoring the evolution of the amplitude of the peaks appearing in the 2D spectra as a function of time allows us to study coherent superpositions of exciton states. Broadband femtosecond pulses can prepare a coherent superposition of excitonic states with well-defined phase that, in turn, causes the amplitude of the peaks of the 2D spectra to oscillate with time T . These oscillations have a frequency corresponding to the difference in energy between the two excited states. Interaction of the system with the surrounding environment causes the optical transition frequencies to fluctuate in time, thus destroying the phase relation in the exciton superposition. This results in exponential damping of the oscillations, which characterizes the dephasing time of the superposition of excited states. In Fig. 3a–c , we show the overall time evolution of the absorptive 2D spectrum (total and real part) of CdSe/CdZnS NPLcs550. Figure 3: Evidence for electronic coherences. ( a – c ) Absorptive 2DES spectra (total and real signal) of CdSe/CdZnS NPLs at four different waiting times ( T shown in inset). The spectra show no obvious differences, except for the upper cross-peak that grows in time, owing to the LX to HX exciton relaxation. ( d , e ) The electronic coherences are revealed by quantum beats along T in the high-energy diagonal peak ( d , blue dots) and in the lower cross-peak ( e , red dots) of the total signal ( T ). The oscillations come from the rephasing pulse sequence (R, black diamonds) for the cross-peak, whereas from the non-rephasing one (NR, grey triangles) in the case of the diagonal peak, as expected for pure electronic coherences. All the time traces correspond to an average of three different experimental scans. ( f , g ) Fourier transforms of the different signals to highlight the frequency spectrum of coherent oscillations. Full size image The amplitude of the higher-energy diagonal peak ( Fig. 3d , blue curve) and lower cross-peak ( Fig. 3e , red curve) are plotted as a function of the waiting time T . Oscillations are evident and visible for ~150 fs in the case of the cross-peak. The frequency of the oscillations in these two peaks (see the Fourier transforms in Fig. 3f,g ) matches the HX–LX frequency difference measured by the absorption spectrum. The non-rephasing signal contributes to the oscillations in the diagonal peak, whereas the cross-peak amplitude oscillates from the rephasing signal only. This is consistent with signatures of electronic coherences [37] , [38] . Phonon modes can be excluded as the source of these oscillations, because the optical and acoustic phonon frequencies in II–VI semiconductor materials are at least one order of magnitude smaller than the HX–LX frequency splitting, as confirmed in pump–probe experiments accessing longer timescales ( Supplementary Fig. 7 and Supplementary Table 5 ). It is not clear why no oscillations can be observed in the two other peaks of the 2D map ( Supplementary Fig. 8 ). This might be due to a larger amplitude of population dynamics contribution, in particular for the upper cross-peak where an exponential growth dominates, owing to the LX to HX exciton relaxation ( Supplementary Fig. 8 ). The oscillating signals in the amplitude of the rephasing pulse sequence at the lower cross-peak were extracted and isolated from the population (incoherent) contribution for three different NPL samples (CdSe NPL550, CdSe/CdZnS NPLcs550 and NPLcs510, another core/shell sample with a thinner core, see Supplementary Figs 9 and 10 ). The real part of the rephasing and non-rephasing signals of CdSe NPL550 and CdSe/CdZnS NPLcs510, with the corresponding Fourier transformations, show similar behaviour than CdSe/CdZnS NPLcs550 ( Supplementary Figs 11 and 12 ). For each sample, the decaying oscillations were fitted with a single exponentially damped sine function, to extract the frequency and dephasing time T 2 ( Supplementary Fig. 13 ). For the three different samples, dephasing times of the HX–LX purely electronic coherence are found to be in the range 15–25 fs. A better fit to the data over longer pump–probe delay times ( T >100 fs) was obtained by adding a small amplitude contribution from a second damped sine function associated with a longer decay time ( Fig. 4a–c and Supplementary Table 6 ). The origin of this additional longer-lived coherence is unclear (see Supplementary Note 5 ). Figure 4: Determination of the excitonic coherence dephasing times. ( a – c ) The amplitude evolutions along the waiting time T of the lower cross peak of the rephasing 2D spectrum (real part and population relaxation removed) of CdSe NPL550 ( a ), CdSe/CdZnS NPLcs550 ( b ) and CdSe/CdZnS NPLcs510 ( c ) are shown as black dots. The error bars, when displayed, are the s.d. estimated from three different scans. Red lines: fits with two exponentially damped sine functions. Parameters relating to the short decay are shown in red (frequency Δ f and dephasing time T 2 ). For each sample, the HX–LX splitting frequency evident from the absorption spectrum shown in the inset of each panel matches the frequency of the coherent oscillation detected by 2DES. Full size image The HX–LX electronic coherence dephases for the three different samples with time constants of 16, 13 and 28 fs for NPL550, NPLcs550 and NPLcs510, respectively. If we assume that dephasing of the LX and HX optical coherences are completely uncorrelated, then the correlation functions for the transition energy gap fluctuations of the exciton superposition state is the sum of the HX and LX energy gap correlation functions ( Supplementary Note 6 ). Using the optical coherence time T 2,HX and T 2,LX of each sample ( Supplementary Table 4 and see Supplementary Fig. 14 for the fit of NPLcs510), the uncorrelated model of dephasing predicts decoherence times for the three samples of 10, 5.4 and 7.4 fs (see Supplementary Fig. 15 , model a). Compared with studies of molecular excitons, there is relatively good agreement between the predictions based on measurements of the optical coherences and the dephasing of the HX–LX exciton electronic coherence (same order of magnitude). However, the longer experimental dephasing times compared with the prediction evidence a partial correlation in the decoherence of HX and LX optical transitions. We use a simple model to rationalize the results between optical and exciton coherence times (model b, Supplementary Fig. 15 ). In this model, the coupling with the phonons leads to similar energy fluctuations of the two excited states. However, the LX transition is additionally broadened by two intrinsic dephasing pathways: from the exciton relaxation to HX (negligible) and through the coupling with the underlying continuum [35] . Following this model, we predict the exciton dephasing time to be ~22, 13 and 20 fs for NPL550, NPLcs550 and NPLcs510, respectively, which is in relatively good agreement with the dephasing times found experimentally. The partial correlation in the HX and LX energy fluctuations explains how the laser power can have a large effect on the optical dephasing without affecting much the exciton coherence. So far, only two research groups have applied 2DES to study colloidal semiconductor nanocrystals. Except one recent publication [33] , no electronic coherence was reported [24] , [39] or only with a very fast decoherence time, that is, with oscillations observable mostly within the pulse duration [27] . From the results, it is evident that the pure homogeneous line broadening of the colloidal NPLs enables clear observation of the electronic coherence that is hidden by inhomogeneous dephasing in the case of the CdSe colloidal quantum dots. CdSe NPLs with perfectly defined thickness is a good system to study pure decoherence without being affected by ensemble disorder. In addition, owing to strong exciton delocalization in the 2D plane of the core/shell NPLs, atomic-scale fluctuations of the thickness of the heterostructure has a minor contribution to the inhomogeneous broadening. A serious issue raised by previous studies of electronic coherence in complex systems has been how to explain the long T 2 times of exciton coherences compared with the short dephasing times of optical coherences. In NPLs, the time scales of the optical and exciton coherences are of the same order of magnitude. However, we find that the narrow spectral lineshapes of the NPLs are not sufficient to explain exciton coherence lasting up to about 100 fs. A partial correlation of energy gap fluctuations underpinning dephasing is found to be important. Molecular systems such as bichromophores can also exhibit transitions with relatively narrow linewidths and superpositions of Frenkel exciton states can be excited. The vibrational motions of molecules, however, play interesting roles in the subsequent dynamical evolution. For example, ultrafast relaxation of the higher-energy exciton to the lowest molecular exciton by radiationless transitions can diphase the exciton superposition [40] . In contrast, vibrations are implicated in sustaining coherence [14] , [15] , [16] . The present work, where vibrational levels are not in resonance with the frequency difference between exciton states and the exciton superposition dephases on the time scale of optical coherences, indirectly lends support to that hypothesis. The clear detection of electronic coherence within a single structure as reported here is therefore a fundamental step towards a deeper understanding of the factors limiting exciton coherence in complex systems at ambient temperature. How to cite this article: Cassette, E. et al . Room-temperature exciton coherence and dephasing in two-dimensional nanostructures. Nat. Commun. 6:6086 doi: 10.1038/ncomms7086 (2015).